Rotating-frame relaxation as a noise spectrum analyser of a superconducting qubit undergoing driven evolution Gate operations in a quantum information processor are generally realized by tailoring specific periods of free and driven evolution of a quantum system. Unwanted environmental noise, which may in principle be distinct during these two periods, acts to decohere the system and increase the gate error rate. Although there has been significant progress characterizing noise processes during free evolution, the corresponding driven-evolution case is more challenging as the noise being probed is also extant during the characterization protocol. Here we demonstrate the noise spectroscopy (0.1–200 MHz) of a superconducting flux qubit during driven evolution by using a robust spin-locking pulse sequence to measure relaxation ( T 1ρ ) in the rotating frame. In the case of flux noise, we resolve spectral features due to coherent fluctuators, and further identify a signature of the 1 MHz defect in a time-domain spin–echo experiment. The driven-evolution noise spectroscopy complements free-evolution methods, enabling the means to characterize and distinguish various noise processes relevant for universal quantum control. Within the gate-based model of quantum computation, a quantum algorithm may be efficiently implemented on a quantum information processor by decomposing it into a finite and discrete set of coherent gate operations [1] . Their realization, although in detail dependent on the particular physical-qubit modality, may be broadly divided into two categories, free evolution and driven evolution, indicating the period(s) during which the desired gate operates on the system. During these two types of evolution, unwanted environmental noise acts to decohere the system and increase the gate error rate. Although process tomography may provide the complete map of the action of a gate operation, it does not characterize the noise sources, which cause fidelity degradation and which, in principle, may differ under free- and driven-evolution conditions. In contrast, the noise sensitivity of the quantum device itself, in conjunction with tailored pulse sequences, may be used to identify spectral features of the noise and thereby elucidate the underlying noise mechanisms [2] , [3] . Dynamical decoupling protocols, for example, spin–echo and its multi-pulse extensions, have been applied to mitigate dephasing during free evolution in numerous qubit modalities, including atomic ensembles [4] , [5] and single atoms [6] , spin ensembles [7] , diamond nitrogen-vacancy centres [8] , [9] , semiconductor quantum dots [10] , [11] , and superconducting qubits [12] . The spectral filtering properties [13] of these and related sequences have proven a useful tool for performing free-evolution noise spectroscopy with superconducting qubits over a wide range of frequencies spanning millihertz [14] , [15] to over 20 MHz [12] . Several groups have also made progress characterizing [12] , [16] , [17] and mitigating [18] decoherence during driven evolution. This case is more difficult in practice, however, because driven-evolution decoherence may be highly correlated with the operational errors that occur while implementing a particular protocol. Such correlations pose challenges for fault-tolerant quantum information processing, and it motivates the importance of characterizing the noise processes that are manifest while the qubit is under external drive. Noise spectroscopy during driven evolution has been studied most extensively via Rabi nutation of the qubit between its ground and excited states, achieved by continuously driving the qubit with an oscillating field. Noise power at the Rabi frequency is inferred from the Rabi-oscillation-decay envelope, and the noise spectrum is reconstructed over the achievable range of Rabi frequencies by varying the field amplitude [12] , [16] , [17] (and F. Yoshihara et al. , manuscript in preparation). There are several drawbacks to this approach, however, including the Rabi experiment’s associated transverse decay, its sensitivity to low-frequency fluctuations of the Rabi frequency, the interpretation of the resultant non-exponential decay law, and the practical consideration of sampling sufficiently many points to resolve and fit accurately a decaying sinusoid oscillating at the Rabi frequency. This type of Rabi-based noise spectroscopy can, however, be generalized by preparing the qubit in an arbitrary initial state. One unique case, originating within the NMR community, is the so-called T 1ρ experiment [16] , [19] , [20] , [21] , [22] , which measures the driven-evolution analogue to T 1 relaxation. In T 1ρ , the driving field is applied along an axis collinear with the qubit’s state-vector in the rotating frame, resulting in a condition called ‘spin locking.’ The main advantages of T 1ρ -based noise spectroscopy are that the qubit decays longitudinally from the spin-locked state with a straightforward exponential decay law (no oscillations); the decay is dominated by noise at the spin-locking frequency and, like its T 1 analogue, is relatively insensitive to broadband low-frequency noise; and it can therefore have higher accuracy over a wider frequency range than the standard Rabi-based approach. In this work, we develop a modified T 1ρ pulse sequence to perform noise spectroscopy during the driven evolution of a superconducting flux qubit. The modified pulse sequence addresses several non-idealities due primarily to 1/f-type noise that may pollute the spin-locking dynamics when using the conventional T 1ρ sequence. Using this improved sequence, we measure both the flux and tunnel-coupling noise spectra during driven evolution over the frequency range 0.1–200 MHz. The observed flux-noise power spectral density (PSD) generally agrees with the 1/ f dependence found independently using free-evolution noise spectroscopy [12] . Notably, between the experiments by Bylander et al. [12] and those presented here, we thermal-cycled the device from 12 mK to 4 K and back again. With the higher accuracy afforded by the T 1ρ measurement, we resolved two additional ‘bump’-like features in the spectrum, possibly due to a set of two-level systems (TLSs), for example, electron spins, that were apparently activated by the thermal cycling. We further demonstrate that the underlying noise mechanisms associated with these particular spectral features are also active during free evolution by observing their signature in a time-domain echo experiment. Device Our test device is a superconducting flux qubit ( Fig. 1a ), an aluminium loop interrupted by four Al-AlO x -Al Josephson junctions. When an external magnetic flux Φ≈Φ 0 /2 threads the loop, the qubit’s potential energy assumes a double-well profile. The wells are associated with clockwise and counterclockwise circulating currents of magnitude I p ≈180 nA and energies ± h ε/2=± I p (Φ−Φ 0 /2) tunable by the applied flux. These diabatic circulating-current states tunnel-couple with a strength Δ=5.4 GHz, and the resulting hybridized qubit states are manipulated using microwave pulses that couple to the qubit via an on-chip antenna. The qubit is embedded in a DC SQUID, a sensitive magnetometer which serves as the qubit readout. The device and measurement set-up is detailed further by Bylander et al. 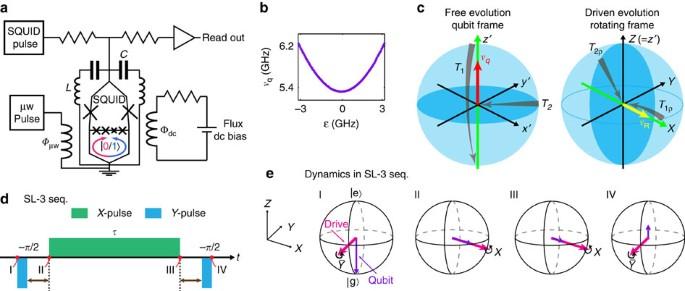Figure 1: Device schematic and spin-locking dynamics. (a) Schematic of the flux qubit with measurement set-up. (b) Measured qubit frequency versus flux bias. (c) Analogy between free and driven evolution. Red and yellow arrows indicate the quantizing field, respectively. The longitudinal axes are highlighted by green arrows, and the transverse planes are highlighted by the blue disks. Grey arrows indicate the temperature-dependent longitudinal (T1andT1ρ) and transverse (T2andT2ρ) depolarization. (d) Standard three-pulse spin-locking sequence (SL-3). Green and blue indicateX- andY-pulse, respectively. (e) Bloch sphere representation of the rotating-frame qubit dynamics under SL-3. The purple arrows are the qubit’s state polarization, while the magenta arrows indicate the driving-field orientation. The qubit is initially prepared in its ground state (I). The firstπ/pulse rotates the qubit by 90° into the equatorial plane (II). The second 90°-phase-shifted continuous driving pulse of durationτ, is then aligned with the qubit state, effectively locking the qubit alongX. During the pulse, the qubit undergoes relaxation in this rotating frame towards its steady state (III). The finalπ/pulse projects the remaining polarization ontoZ(=z′) for readout (IV). [12] Figure 1: Device schematic and spin-locking dynamics. ( a ) Schematic of the flux qubit with measurement set-up. ( b ) Measured qubit frequency versus flux bias. ( c ) Analogy between free and driven evolution. Red and yellow arrows indicate the quantizing field, respectively. The longitudinal axes are highlighted by green arrows, and the transverse planes are highlighted by the blue disks. Grey arrows indicate the temperature-dependent longitudinal ( T 1 and T 1ρ ) and transverse ( T 2 and T 2ρ ) depolarization. ( d ) Standard three-pulse spin-locking sequence (SL-3). Green and blue indicate X - and Y -pulse, respectively. ( e ) Bloch sphere representation of the rotating-frame qubit dynamics under SL-3. The purple arrows are the qubit’s state polarization, while the magenta arrows indicate the driving-field orientation. The qubit is initially prepared in its ground state (I). The first π / pulse rotates the qubit by 90° into the equatorial plane (II). The second 90°-phase-shifted continuous driving pulse of duration τ , is then aligned with the qubit state, effectively locking the qubit along X . During the pulse, the qubit undergoes relaxation in this rotating frame towards its steady state (III). The final π / pulse projects the remaining polarization onto Z (= z ′) for readout (IV). Full size image Reference frames and Hamiltonians In the laboratory frame and within a TLS approximation, the qubit Hamiltonian is: where and are Pauli operators. δ Δ( t ) and δ ε( t ) represent random fluctuations in the effective tunnel-coupling and flux terms, respectively, and the oscillating term represents the harmonic driving field that is treated semiclassically with amplitude A rf ( t ), frequency v rf and phase φ . Although noise affecting the qubit physically manifests itself in the lab frame (equation 1), the longitudinal ( T 1 and T 1ρ ) and transverse ( T 2 and T 2ρ ) relaxation times for free- and driven evolution may be analogously defined in the qubit-eigenbasis and rotating frames, respectively, as described below and presented in Table 1 (also see Supplementary Note 1 and Supplementary Table S1 for detailed derivation and description). Their measurement may then be related back to the physical noise parameters in the laboratory frame. Table 1 Comparison of decohering properties of a flux qubit during free and driven evolution. Full size table Decoherence during free evolution is described by transforming equation 1 to the qubit’s energy eigenbasis: where θ =arctan( ε /Δ) is the rotation angle of the quantization axis from the lab frame, and v q = is the qubit’s frequency splitting ( Fig. 1b ). The standard longitudinal ( T 1 ≡1/Γ 1 ) and transverse ( T 2 ≡1/Γ 2 ) relaxation times are defined in this frame. In our device, T 1 ≈12 μs with only a weak dependence on ε , whereas T 2 ≈3 μs at ε =0 and decreases away from this point [12] . Decoherence during driven evolution (that is, during a constant-amplitude pulse, A rf ( t )= A rf ) is described by a second transformation, taking equation 2 to a reference frame rotating at the drive frequency v rf (omitting stochastic terms): where Δ v=v q − v rf is the frequency detuning between the qubit and the driving field, and v R = A rf cos θ is the Rabi frequency under resonant driving (Δ v =0). Here the rotating wave approximation has been invoked by omitting the fast oscillating terms (see Supplementary Note 1 for a generalization). Analogy between free and driven evolution For resonant driving along the x axis (Δ v =0, φ =0), the Hamiltonian in equation 3 describes a pseudospin quantized along X with a level splitting equivalent to the Rabi frequency v R . The qubit’s Bloch vector precesses around the x axis at a rate v R , and its subtended angle depends on the initial state. That is, the driven evolution of the qubit state may be interpreted as the ‘free evolution’ of a pseudospin around a static field v R ( Fig. 1c ). By analogy with the conventional free-evolution T 1 and T 2 times, we define longitudinal and transverse depolarization times T 1ρ and T 2ρ for the pseudospin with respect to this new quantization axis (see Table 1 ). Just as T 1 depends on the noise at the qubit frequency v q that is transverse to the z ′ axis (equation 2), so is T 1ρ determined by the noise at the pseudospin’s level splitting v R that is transverse to the x axis (equation 3). For completeness, the measurement and value of the rotating-frame decoherence time T 2ρ (‘free-induction’ time in the rotating frame) is equivalent to the conventional Rabi experiment and associated decay time T Rabi ( Supplementary Fig. S2b ). More detailed discussion about the analogy between free evolution and driven evolution in the rotating frame can be found in Supplementary Note 1 . The connection between the driven-evolution times ( T 1ρ , T 2ρ ), the free-evolution times ( T 1 , T 2 ) and the PSD of the physical noise terms (δΔ( t ), δε( t )) is formally made using the generalized Bloch equations [23] , [24] and the transformations between equations 1, 2, 3. The exponential relaxation rate during weak and resonant driving is where stands for the symmetrized PSD of λ -noise, and λ ϵ{Δ,ε… or x ′, y ′, z ′…} indicates either the fluctuating part of the system Hamiltonian or the axis along which those fluctuations occur. The relaxation rate Γ 1ρ arises from two terms related to noise in the qubit-eigenbasis (equation 2). The first term (Γ 1 term) is associated with transverse noise along the x ′ axis at frequency v q ± v R (which appears as v R in the rotating frame). The second term (Γ v term) is the longitudinal noise along the z ′ axis at the drive frequency v R , which is directly transferred into the rotating frame. This latter term provides a direct method to extract the noise PSD at the locking Rabi frequency by measuring relaxation during driven evolution via a T 1ρ experiment. Advantages of T 1ρ over Rabi spectroscopy The T 1ρ experiment, when utilized as a noise spectrum analyser to extract the PSD, has inherent advantages over direct Rabi-based techniques [12] , [17] (and F. Yoshihara et al. , in preparation). One major shortcoming of the Rabi method is its vulnerability to low-frequency fluctuation δv R of the effective Rabi frequency. First, the Rabi frequency is first-order sensitive to fluctuations of the driving-field amplitude δv R (proportional to δA rf ), whose RMS fluctuation is found in this case proportional to v R ( δv R ≈0.06% v R ) [18] . Hence, the temporal v R inhomogeneity becomes important when the driving is strong (large v R ). In addition, low-frequency fluctuation of the qubit’s level splitting ( δv ) modulates the effective Rabi frequency to second order, adding to the inhomogeneous broadening [12] . The effect dominates the Rabi decay when the driving is weak enough (small v R , as the second-order contribution / v R exceeds decay rates from other sources) ( Table 1 ). These two effects are analogous to the scenarios of free-evolution dephasing due to low-frequency noise via linear and quadratic coupling, respectively [16] . In contrast, the locking dynamics in the T 1ρ experiment largely reduce its sensitivity to these fluctuations, and thus substantially improves the accuracy of the extracted noise PSD, especially at both high and low-frequency regimes. In addition, T 1ρ has a simple exponential decay law, whereas the Rabi decay law can be complicated by its sinusoidal nutation in conjunction with a non-exponential decay envelope related to its sensitivity to low-frequency noise (see Table 1 ), both of which pose a challenge to high-precision fitting. A T 1ρ measurement requires far fewer datapoints than would a Rabi decay envelope on a sinusoid oscillating at the Rabi frequency. These properties make the T 1ρ method more accurate and experimentally efficient. Conventional T 1ρ sequence The measurement of the rotating-frame relaxation time T 1ρ begins by preparing the qubit state to be either parallel or anti-parallel with X (collinear with the driving field), corresponding to the pseudospin’s ground and excited state, respectively. This results in the so-called ‘spin-locking’ condition, a reference to the pseudospin remaining aligned in the absence of noise with the static driving field v R in equation 3 (see Fig. 1e and Supplementary Fig. S2a ). The measurement of the relaxation time from the spin-locked condition to a depolarized steady-state is the so-called T 1ρ experiment. The original T 1ρ sequence as developed in NMR and applied to superconducting qubits was a three-pulse sequence [25] , two π /2 pulses separated by a 90°-phase-shifted continuous driving pulse (labelled here ‘SL-3’, see Fig. 1d ). The phase shift is implemented by altering the driving-field phase φ via standard IQ-mixing techniques. The dynamics can be visualized with the assistance of the Bloch sphere within the rotating frame ( Fig. 1e ). For convenience, we use { X , Y , Z } to denote rotating-frame coordinates, pulse phase and qubit states. The first pulse (bar indicates negative or 180-degrees-rotated orientation) brings the qubit from its ground state to the equator, parallel with X (step I). The driving field is then applied along X and thereby aligned with the qubit state, so that the qubit is effectively locked in this orientation and experiences relaxation Γ 1ρ only (steps II and III). After a finite duration τ , the remaining polarization along X is projected, by the last pulse, back along Z for readout (step IV). The long-time, steady-state population carries no net X -polarization, because the device is operated in the limit v R << k B T / h =1.3 GHz, where T ≈65 mK is the effective device temperature obtained by measuring the SQUID’s switching-current distribution. The – X – phase order applied here and the X – Y – X one by Collin et al. [25] are effectively the same, as only the relative phase is important. We repeat the same sequence on a nominally identically prepared system a few thousand times to improve state estimation. Hence, decoherence of this system should be understood in the sense of a temporal ensemble average. Modified T 1ρ sequence In solid-state systems, the recorded T 1ρ decay signal using the original (SL-3) sequence may suffer from several types of system imperfection, in particular, signal distortion due to low-frequency noise via other channels. One example of a measured T 1ρ trace is shown in Fig. 2b (brown trace). Another example can be found in the studies of Collin et al. [25] , an early demonstration of spin-locking implemented on a quantronium qubit. A prominent feature in these examples is the presence of unwanted Rabi-frequency oscillations on the back of an otherwise exponential decay function. We excluded the possibility of a constant frequency detuning in our experiment, which could effectively separate the driving field and qubit state during the locking period and lead to oscillations. Rather, we determined that the oscillations were due to dephasing during the intervals between adjacent pulses. In our experiments, we use Gaussian pulses with ~10 ns width for the π /2 pulses and Gaussian rise-and-fall for the long driving pulse. To clearly separate pulses, there is a practically unavoidable duration of free evolution between pulses ( Fig. 1d ). Depending on the length τ of the second pulse, phase diffusion accumulated during the first interval will sometimes be doubled (for v R τ =1,2,3…), and sometimes be refocused (for v R τ = , 1 , 2 …), producing those oscillations. In the presence of this noise, the locking protocol is compromised to a differing degree for the temporal ensemble elements, making the observed decay a complicated combination of precession, relaxation and decoherence processes. To correct for it, we developed a modified five-pulse sequence (labelled ‘SL-5a,’ see Fig. 2a ), which adds one π X pulse in the middle of each interval in SL-3. The added pulses refocus the phase diffusion as is done in a spin–echo sequence [26] . Relaxation obtained using SL-5a is shown in Fig. 2b , and it shows a clear improvement (no oscillation) over SL-3. 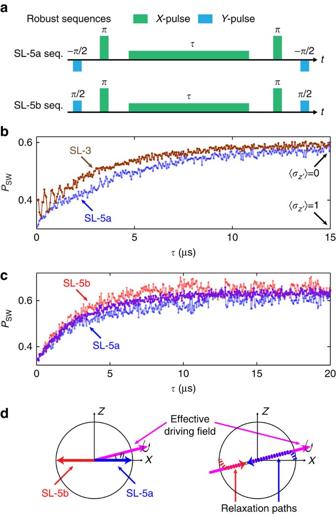Figure 2: Robust spin-locking sequences. (a) Modified five-pulse sequences (SL-5a and SL-5b), robust in the presence ofδεandδΔ low-frequency noise. (b) Comparison of measured signals by SL-3 (brown) and SL-5a (blue). Both traces are taken atε=192 MHz andvR=3 MHz.PSWis the measured switching probability of the readout SQUID, and is linear with the qubit’s state population. (c) Comparison of measured signals by SL-5a (blue), SL-5b (red) and their average (purple). Both traces are taken atε=960 MHz andvR=24 MHz. The data are taken in an interleaved order between blue and red traces. (d) Cross-section sketch of the qubit dynamics under the SL-5a and SL-5b protocols, with the driving field (magenta arrow) tilted by an angleη(η>0 in this example) due to slow fluctuations of the frequency detuning. On the left are the qubit states right before the locking pulse; on the right, their relaxation paths during the locking period are indicated by the dashed lines. The steady-state solution (the contacting point of blue and red dash lines) deviates away from=0 whenη≠0. Figure 2: Robust spin-locking sequences. ( a ) Modified five-pulse sequences (SL-5a and SL-5b), robust in the presence of δε and δ Δ low-frequency noise. ( b ) Comparison of measured signals by SL-3 (brown) and SL-5a (blue). Both traces are taken at ε =192 MHz and v R =3 MHz. P SW is the measured switching probability of the readout SQUID, and is linear with the qubit’s state population. ( c ) Comparison of measured signals by SL-5a (blue), SL-5b (red) and their average (purple). Both traces are taken at ε =960 MHz and v R =24 MHz. The data are taken in an interleaved order between blue and red traces. ( d ) Cross-section sketch of the qubit dynamics under the SL-5a and SL-5b protocols, with the driving field (magenta arrow) tilted by an angle η ( η >0 in this example) due to slow fluctuations of the frequency detuning. On the left are the qubit states right before the locking pulse; on the right, their relaxation paths during the locking period are indicated by the dashed lines. The steady-state solution (the contacting point of blue and red dash lines) deviates away from =0 when η ≠0. Full size image In several measured traces, we observe a second type of signal distortion—random fluctuations at the few-percent level on the exponential signal, and at a time scale of minutes or tens of minutes—for example, Fig. 2c (blue trace). As we describe in detail below, low-frequency fluctuations of the frequency detuning result in the ‘shivering’ of the effective Rabi field and, thereby, fluctuations in the observed decay signal. We first describe how we corrected the distortion, and then explain its origin. The solution is to use a complementary pulse sequence (labelled ‘SL-5b,’ see Fig. 2a ) together with SL-5a. The new sequence is nominally identical to SL-5a, except that we replace the two pulses with two π /2 Y pulses, such that the qubit Bloch vector is anti-parallel with the driving axis for SL-5b. Ideally, both sequences should give the same decay function. However, when we apply the sequences in an interleaved sampling order (inner loop: alternate between SL-5a and SL-5b; outer loop: step τ ), the anti-symmetry of the signal fluctuation, slow compared with the collection time at each value τ , is captured by the twin sequences, as shown by the example in Fig. 2c . We then recover the smooth exponential decay by taking the average of the two traces. Our ability to recover a smooth exponential decay is closely related to the ultra-slow (~minutes) fluctuation of frequency detuning δv . First, the occurrence of the signal distortion at large τ indicates a deviation of the steady-state population from zero X -polarization. Assuming small detuning (Δ v << v R ), to first order, the steady-state X -polarization [24] (and Supplementary Note 1 ), in the practical limit v R << k B T / h << v q , is where η =arctan(Δ v / v R ) is the angle of the driving field with respect to X due to frequency detuning (see Fig. 2d ). Equation 6 is applicable to both SL-5a and SL-5b, but the difference in the last back-projection pulse gives rise to a differential signal response to the non-zero X -polarization. Therefore, fluctuation of the frequency detuning, to first order, causes fluctuation of the steady-state longitudinal polarization and the anti-symmetric feature of the traces in Fig. 2c . The relaxation dynamics in both sequences with finite detuning are sketched in the right panel of Fig. 2d . Ignoring the process at small τ where the much faster T 2ρ process is involved, the normalized decay signal, to first order of η , can be approximated as P a ( τ )= for SL-5a, and P b ( τ )= for SL-5b. The average P ( τ )= becomes independent of detuning, and recovers the underlying relaxation signal. Noise spectroscopy during driven evolution We use the modified T 1ρ pulse sequence to implement noise spectroscopy during driven evolution ( Fig. 3 ). To derive the Δ-noise PSD, we perform a driven-evolution T 1ρ measurement for various v R at ε =0, where the qubit is first-order insensitive to ε noise, as well as the standard (free-evolution) inversion-recovery T 1 -measurement [26] . Both T 1 and T 1ρ traces are fit to extract the exponential decay rates Γ 1 and Γ 1ρ , which give the Δ-noise PSD by S Δ ( v R )= S z′ ( v R )=2Γ 1ρ −Γ 1 . For ε -noise PSD, we perform the same experiments at ε ≠0, where the qubit becomes predominantly sensitive to ε noise. We then have S ε ( v R )=[ S z′ ( v R )−cos 2 θS Δ ( v R )]/sin 2 θ =[2Γ 1ρ −Γ 1 −cos 2 θS Δ ( v R )]/sin 2 θ , where S Δ ( v R ) is previously measured. The locking Rabi frequency, v R , is determined by measuring Rabi oscillations with the same driving-field amplitude. The lower limit (~100 kHz) of the spectrum is determined by the Δ v inhomogeneity , which breaks the locking condition when driving is too weak. On the other hand, an undetermined effect (presumably heating due to strong driving), which distorts the SQUID’s switching-current distribution, prevents us from probing higher frequency than ~200 MHz. We believe the limitation is unrelated to the SQUID plasma mode, which is around ~2.3 GHz for this device. 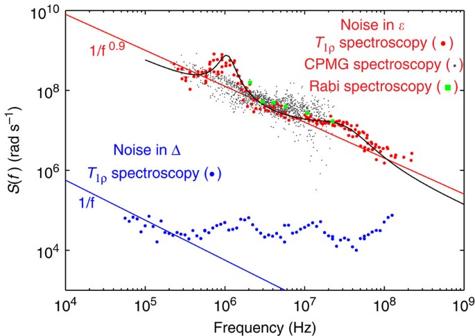Figure 3: Noise spectroscopy during driven evolution. ε(red dots) and Δ (blue dots) noise spectroscopy by theT1ρmethod. Here, previous results onεnoise by the CPMG (grey dots) and Rabi (green squares) methods measured on the same device are plotted for comparison. From the fitting results, the error rate in the worst case is about 30% forεnoise, and 70% for Δ noise. Previous experiments and theT1ρexperiment were separated by 6 months and a 4-K warm-up. The red and blue solid lines are the 1/fαpower laws, extrapolated from separate low-frequency noise measurements14. The black line represents the functionS′(f)=A/f0.9+S1(f;F1,W1)+S2(f;F2,W2), where (f;F,W)=W2/((f−F)2+W2), andA=(2π0.65 × 106)2(rad s−1)2,S1=7.0 × 108rad s−1,F1=1.05 MHz,W1=0.25 MHz,S2=1.2 × 107rad s−1,F2=20 MHz,W2=25 MHz. Figure 3: Noise spectroscopy during driven evolution. ε (red dots) and Δ (blue dots) noise spectroscopy by the T 1 ρ method. Here, previous results on ε noise by the CPMG (grey dots) and Rabi (green squares) methods measured on the same device are plotted for comparison. From the fitting results, the error rate in the worst case is about 30% for ε noise, and 70% for Δ noise. Previous experiments and the T 1 ρ experiment were separated by 6 months and a 4-K warm-up. The red and blue solid lines are the 1/ f α power laws, extrapolated from separate low-frequency noise measurements [14] . The black line represents the function S ′( f )= A / f 0.9 + S 1 ( f ; F 1 , W 1 )+ S 2 ( f ; F 2 , W 2 ), where ( f ; F , W )= W 2 /(( f − F ) 2 + W 2 ), and A =(2 π 0.65 × 10 6 ) 2 (rad s −1 ) 2 , S 1 =7.0 × 10 8 rad s −1 , F 1 =1.05 MHz, W 1 =0.25 MHz, S 2 =1.2 × 10 7 rad s −1 , F 2 =20 MHz, W 2 =25 MHz. Full size image In this device, the measured Δ-noise spectrum is generally white. As the extrapolated 1/ f Δ-noise from low-frequency measurements crosses the white noise level around the lower limit, we are unable to determine whether the 1/ f noise extends to this regime or has a cutoff [14] . The noise could be due to Johnson noise from charge or critical current fluctuations, or due to thermal photon noise [27] originating from the LC resonator associated with the readout SQUID, which inductively couples to the qubit ( Fig. 1a ). The ε -noise spectrum exhibits a 1/ f α dependence with α =0.9, a value that generally agrees with independently measured free-evolution noise spectroscopy using a Ramsey (1 mHz–100 Hz) [14] and Carr–Purcell–Meiboom–Gill (CPMG; 0.1–20 MHz) approach [12] . Although not necessarily a universal result, this suggests that driven evolution does not activate ε -noise sources for this device. In general, the T 1ρ spectroscopy confirms these results with better accuracy and extends the frequency range by 5x (presumably limited in this device by a heating effect at high driving fields). Note that measuring at higher frequency (0.1–1 GHz) is feasible in principle by using this technique. Spectral and temporal signatures of coherent TLSs In contrast to previous free-evolution measurements, we observe on the 1/ f trend two clear ‘bump-like’ features, one around 1 MHz and the other around 20 MHz. These features appeared after thermal-cycling the device from base temperature to 4.2 K and back again, which likely activated the fluctuators. The one at 1 MHz has a clear peak above the general 1/ f background. This excludes the possibility of random telegraph noise (RTN), possibly generated by some microscopic two-level fluctuators, as the cause of this bump, as RTN would produce a Lorentzian spectrum centred at zero frequency [28] , [29] . To fit the main features, we assume that the ε -noise PSD is a combination of the 1/ f 0.9 line and two Lorentzians. Both bumps are better fit to Lorentzians centred around 1 and 20 MHz than those centred at zero frequency. One example is shown by the black line in Fig. 3 . We find a signature of the 1 MHz bump feature in a free-evolution, time-domain echo experiment. 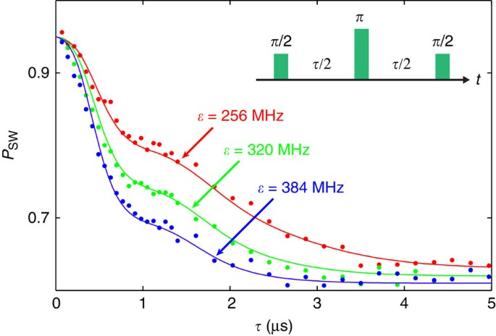Figure 4: Temporal signature of TLS during free-evolution. Echo phase-memory decay (dots) measured atε=256 MHz (red), 320 MHz (green) and 384 MHz (blue), and corresponding simulation (solid lines) with assumed flux-noise PSD function,S′(f)=A/f0.9+S1L(f;F1W1), whereA=(2π0.9 × 106)2(rad s−1)2,S1=9.0 × 108rad s−1,F1=1.25 MHz,W1=0.35 MHz. The temporal signature of the Lorentzian at 1 MHz is essentially independent of theεbias. Inset is the echo pulse sequence. Here,τis the total free evolution time in the sequence. Note that the 20 MHz bump has little influence at these bias points. Figure 4 shows the spin–echo phase-decay as measured at several flux-bias points where the qubit coherence is mostly limited by ε noise. Under a Gaussian-noise assumption, the echo sequence is most sensitive to the noise whose frequency is about the inverse of the total free-evolution time of the sequence. The echo-decay functions all exhibit a clear ‘dip’ feature around 1 μs, corresponding to the spectral feature around 1 MHz. To model this result, we use the previously assumed PSD function S ′( f ) (1/ f 0.9 plus two Lorentzians) with tunable parameters to reproduce the echo-decay signal by the filter function method [12] , [16] , [30] . The agreement is good, and bump parameters estimated from the temporal echo measurement are within 30% of a direct fit to the driven-evolution spectral data. In general, we are able to predict the phase decay from the T 1ρ spectroscopy results, and, in turn, justify the performance of the T 1ρ spectroscopy method on a superconducting qubit. In the case of the 20-MHz Lorentzian, simulations indicate that the echo signature corresponding to this broad, relatively small feature in the noise spectrum would yield only a small deviation from the spin–echo phase-decay function with no discernable ‘dip.’ The temporal resolution in Fig. 4 is furthermore insufficient to resolve such a deviation. We note that on a subsequent cooldown, with the qubit exhibiting a similarly small spectral feature, we did observe a small distortion (but no ‘dip’) in the expected spin–echo phase-decay function. Figure 4: Temporal signature of TLS during free-evolution. Echo phase-memory decay (dots) measured at ε =256 MHz (red), 320 MHz (green) and 384 MHz (blue), and corresponding simulation (solid lines) with assumed flux-noise PSD function, S ′( f )= A / f 0.9 + S 1 L ( f ; F 1 W 1 ), where A =(2 π 0.9 × 10 6 ) 2 (rad s −1 ) 2 , S 1 =9.0 × 10 8 rad s −1 , F 1 =1.25 MHz, W 1 =0.35 MHz. The temporal signature of the Lorentzian at 1 MHz is essentially independent of the ε bias. Inset is the echo pulse sequence. Here, τ is the total free evolution time in the sequence. Note that the 20 MHz bump has little influence at these bias points. Full size image It is possible that the observed Lorentzian bumps are generated by two sets of coherent TLSs [31] , such as electron spins. In a magnetic environment, each spin executes Larmor precession at a frequency proportional to its local field. Its transverse component couples to the qubit’s flux degree of freedom with a strength depending on geometric relations among the device, the field and the spin [32] , and adds to a net fluctuating flux whose PSD reflects the spectral (Larmor frequency) distribution of spins, even though the ensemble has already lost its coherence. The width of the Lorentzian indicates in part the field inhomogeneity. Assuming uncorrelated surface electron spins and an average coupling strength of 2.7 × 10 −8 Φ 0 · from simulation, both Lorentzian bumps correspond to ~10 6 spins. The number scales down in the presence of a high degree of spin order [33] . Moreover, if we assume the spins feel the same magnetic field as the qubit, about 0.5 mT ( B 0 =Φ/ A L , where Φ=Φ 0 /2 is the flux through the qubit loop and A L ≈2 μm 2 is the loop size), the corresponding electron-spin Larmor frequency is 14 MHz. This is only a rough estimate, as screening due to superconducting metal may lead to a large variation of the field at various locations in the vicinity of the metal surface, and other locations for these spins, for example, the superconductor-insulator boundary [34] and substrate, are also possible. Nonetheless, the crude estimate is consistent with our observations. The modified T 1ρ method presented here, in conjunction with existing free-evolution spectroscopy methods, enables the characterization of the noise sources relevant for both driven- and free-evolution quantum control methods. Although many noise sources may be manifest similarly during both conditions, in principle, the noise in these two cases need not be identical. For example, driven evolution may activate certain noise sources that are otherwise dormant during free-evolution. In this demonstration with a flux qubit, the flux and tunnel-coupling noise spectra reveal more detailed information and cover a wider frequency range, a 10 × increase in this device, as compared with our previous free-evolution (CPMG spectroscopy) and driven evolution (Rabi spectroscopy) methods [12] . We observed the spectral features of two sets of coherent TLSs in the environment, possibly due to effective electron spins on the metal surface, which are active during driven evolution. We could furthermore observe a temporal signature of one of these fluctuators in a free-evolution echo experiment, indicating that it is active during both driven and free evolution. This type of noise characterization serves as an important step towards the engineered mitigation of decoherence through improved materials, fabrication, control sequences and qubit design. Our modifications to the T 1ρ pulse sequence target the unwanted effects of low-frequency noise, opening this method to the multiple qubit modalities that are subject to such noise. Description of the qubit We fabricated our device at NEC, using the standard Dolan angle-evaporation deposition process of Al–AlO x –Al on a SiO 2 /Si wafer. Our persistent-current qubit [12] , [35] consists of a superconducting loop with diameter d ~2 μm, interrupted by four Josephson junctions. Three of the junctions each have the Josephson energy E J = h × 210 GHz, and charging energy E C = h × 4 GHz; the fourth is smaller by a factor α =0.54. The qubit is embedded in a hysteretic DC SQUID, a sensitive magnetometer, which is used for the qubit readout. It has a critical current I c,sq =4.5 μA; normal resistance R N =0.25 kΩ; mutual qubit–SQUID inductance M Q–S =21 pH; on-chip shunt capacitors C sh ≈10 pF, inductors L sq ≈0.1 nH, and bias resistors R I =1 kΩ and R V =1 kΩ. The shunt capacitors bring the plasma frequency down to f p =2.1 GHz, which is much higher than the frequencies of the coherent fluctuators presumably related to the frequency- and time-domain results. Pulse generation and calibration The r.f. microwave pulses are created by mixing the in-phase and quadrature pulse envelopes, generated by a Tektronix 5014 Arbitrary Waveform Generator, with a continuous wave, provided by an Agilent E8267D PSG Vector Signal Generator. We use the internal I/Q mixer of the PSG for the envelope mixing. All pulses are further gated in order to eliminate leakage. Imperfections in the electronics and coaxial cables will cause pulse distortions, especially for short pulses (a few nanoseconds long). To ensure that the pulses we send to the cryostat are free from distortions, we first determine the transfer function H ext with a high-speed oscilloscope, and then use to correct for imperfections in the arbitrary waveform generator and in the I/Q mixers [36] . This set-up allows us to create well-defined Gaussian-shaped microwave pulses with pulse widths as short as 2.5 ns. How to cite this article: Yan, F. et al. Rotating-frame relaxation as a noise spectrum analyser of a superconducting qubit undergoing driven evolution. Nat. Commun. 4:2337 doi: 10.1038/ncomms3337 (2013).